Adopting kin enhances inclusive fitness in asocial red squirrels Orphaned animals benefit from being adopted, but it is unclear why an adopting parent should incur the costs of rearing extra young. Such altruistic parental behaviour could be favoured if it is directed towards kin and the inclusive benefits of adoption exceed the costs. Here, we report the occurrence of adoption (five occurrences among 2,230 litters over 19 years) in asocial red squirrels ( Tamiasciurus hudsonicus ). Adoptions were always between kin, while orphans without nearby kin were never adopted. Adoptions were confined exclusively to circumstances in which the benefits to the adopted juvenile ( b ), discounted by the degree of relatedness between the surrogate and the orphan ( r ), exceeded the fitness costs of adding an extra juvenile to her litter ( c ), as predicted by Hamilton's rule ( rb > c ) for the evolution of altruism. By focusing on adoption in an asocial species, our study provides a clear test of Hamilton's rule that explains the persistence of occasional altruism in a natural mammal population. When J.B.S. Haldane was asked whether he would lay down his life to save his brother, he famously replied 'No, but I would to save two brothers or eight cousins' [1] . More formally, Hamilton's rule states that altruism should evolve when the fitness cost to the actor ( c ) is less than the fitness benefit to the recipient ( b ) multiplied by their coefficient of relatedness ( r ) [2] . As a result, providing costly assistance to another individual is likely only when the two individuals are closely related. Adoption (the act of solely and completely caring for another female's offspring as your own until weaning) is often cited as an example of altruism and has been reported in at least 62 mammal species. Most of these cases are among cooperatively breeding and/or highly social species in which groups consist of kin [3] . Although many of these studies put their findings in the context of Hamilton's rule, none have actually been able to calculate the fitness cost to the actor ( c ) in these circumstances [4] , [5] . Fitness costs to the adopting parent are often confounded with potential benefits such as increased survival, rank or reproductive success through effects on group size and social relationships brought about by adopting any individual, even unrelated orphans [6] , [7] . In addition, given that most social groups normally consist of closely related individuals, there is often no opportunity for non-kin to be adopted [4] . These confounding factors would not be present in asocial species, but the three reported cases of adoption by asocial species have all been attributed to misdirected care rather than kin selection [8] . Here, we report instances of adoption in an asocial mammal, for which we can directly quantify all components of Hamilton's rule. We found that orphans were always adopted by closely related kin, despite the odds favouring adoption by unrelated females. Adopting females increased their inclusive fitness because the benefits gained by adopting one closely related orphan outweighed the survival costs to the litter incurred by adding an additional individual. We also observed instances in which orphaned young were not adopted, but the potential surrogate mothers in these cases were not closely related enough to the orphans for the indirect fitness benefits to outweigh the costs of adoption. Together, these findings provide strong empirical support for Hamilton's rule. The asocial nature of red squirrels Individual red squirrels ( Tamiasciurus hudsonicus ) ( Fig. 1 ) defend food-based territories year round using territorial vocalizations [9] , [10] . Removal experiments of territory owners show that squirrels quickly recognize the absence of a neighbour [11] , yet behavioural observations clearly show the lack of physical interactions between adults. Between 1989 and 2008, we have recorded 54,785 red squirrel behaviours and only 307 (0.6%) were classified as physical interactions between adults (excluding male–female matings, dam–offspring and sibling interactions before dispersal from the natal territory). All of these interactions were aggressive territorial chases against intruders. 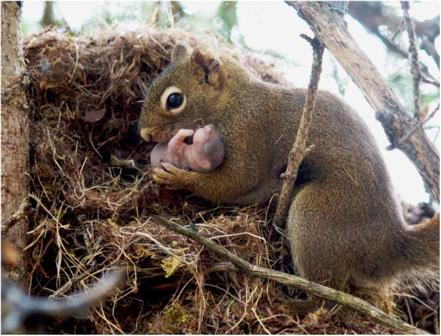Figure 1 Female red squirrel prepares to move a juvenile between nests. Figure 1 Female red squirrel prepares to move a juvenile between nests. Full size image Cases of adoption During detailed study of red squirrels at a single site over the past 19 years (2,230 litters), we have detected five instances of adoption (a lactating dam nursing another dam's juvenile until weaning), for which we knew the ancestry of the dam and the adopted juvenile. These adoptions occurred in different years with different females, but always involved the adoption of kin ( Table 1 ). Four adoptions occurred when the juveniles were between 43 and 63 days old. The individuals (identified by unique ear tags) were seen nursing from and/or nesting with the surrogate dam and her offspring. Nest emergence occurs between 42 and 65 days of age, whereas weaning occurs at 70 days of age [12] , [13] . The fifth adoption was detected when we entered a nest to find one juvenile that was unusually large relative to its littermates (20.6 vs. 13.7 g±0.7 s.e.m.). The mass, sex and presence of an ear notch (juveniles are marked with ear notches just after birth) suggested that the large juvenile originated from a neighbouring litter that had been born and sampled 6 days earlier. This was confirmed using tissue samples collected from both litters, which included identical genotypes across 16 microsatellite loci [14] between this larger juvenile and one of the offspring from the previously sampled litter. This juvenile also mismatched the surrogate dam at three loci, but at none with the original dam. To confirm that identical genotypes were not from different individuals, we used the software package Cervus 3.0 [15] to determine the probability of identical genotypes using allele frequencies estimated from 100 adults from the same grid and year. The probability of another individual matching this genotype was small (1.17×10 −19 ), whereas the probability that a full sibling would have this identical genotype remained unlikely (4.90×10 −7 ). Both these probabilities were smaller than the average probabilities of identity across all genotypes in the population (1.93×10 −17 and 5.20×10 −7 , respectively). As a 6-day-old juvenile would have to be carried to a new nest, we parsimoniously assumed that the surrogate female initiated the adoption rather than the orphaned juvenile. Table 1 Probability and inclusive fitness of adopting kin. Full size table Relatedness of adopted juveniles and surrogates As we knew the maternal ancestry of all squirrels born within our study area, we were able to estimate the minimum relatedness between the surrogate dam and the adopted juvenile using the maternal pedigree in all cases ( Table 1 ). We consider this a minimum degree of relatedness, because our maternal pedigree could not identify individuals related through paternal lineages. We define non-kin to be individuals who were related less than 0.125 through our maternal pedigree. Four cases of adoption occurred in years before we began collecting tissue samples for paternity analyses, whereas the fifth case occurred as we began sampling both adults and juveniles. In this latter case, the maternal pedigree confirmed that the adopted juvenile and surrogate dam were non-uterine siblings ( r ≥0.25). Still, we used the software package SPAGeDi 1.3 [16] to calculate their coefficient of relatedness based on genetic similarity at 16 microsatellite loci [14] , [17] . Here, we present the Queller and Goodnight [18] estimator, which was calculated using allele frequencies estimated from 100 adults from the same grid and year, although other relatedness estimators produced comparable results. The original dam and adopted juvenile were highly related as expected ( r =0.560±0.099; standard error derived from jackknife resampling over loci), whereas the surrogate dam and adopted juvenile were also highly related ( r =0.368±0.158). One-sample t -tests revealed that both of these estimates were significantly greater than zero ( t =5.65, d.f.=15, P <0.00003; t =2.33, d.f.=15, P <0.02, respectively). Adoption and kinship In all adoption cases, the original and surrogate dams occupied territories ≤75 m apart (measured from centre of territories) and gave birth within 19 days of each other. We used these two search criteria to identify potential surrogates and cases in which adoption could occur through the death of one of the lactating females. In the five cases of adoption, the number of potential surrogates surrounding each adopted litter ranged from two to four females, with only one female being kin ( r ≥0.125) in each case ( Table 1 ). We calculated the probability of the litter being adopted by kin based on the proportion of potential surrogates made up by kin. The probability of all five adoptions being by kin was only 1.0%. We identified 29 additional litters in which a dam died and a surrogate was available, but no adoption occurred. In only two of these 29 cases were kin females available to adopt orphaned litters, indicating a strong relationship between adoption and kinship (exact logistic regression odds ratio=56.3, 95% confidence interval 6.2 to unknown, P <0.0002). Testing Hamilton's rule ( rb > c ) Adopting additional juveniles is expected to decrease the surrogate dam's direct fitness, as juvenile survival declines with increasing litter size ( Fig. 2 ) [9] . We determined the relationship between litter size and annual reproductive success (ARS) using 19 years of data for our study population. The fitness cost to the surrogate dam of adoption ( c ) was represented by the reduction in survival of her natal litter, as a result of litter size being increased by one juvenile. The benefit to the adopted juvenile ( b ) was its probability of survival, given the size of its new litter. We then determined the minimum relatedness ( r ) necessary between the surrogate dam and the adopted juvenile for the benefits of adoption to outweigh the costs according to Hamilton's rule ( Fig. 2 ). In all five cases of adoption, surrogate dams were sufficiently related to their adopted juveniles to enhance inclusive fitness, whereas in the two cases when a kin neighbour was present and lactating but did not adopt, adoption would have reduced the female's inclusive fitness ( Table 1 ). Although we were unable to confirm the availability of multiple offspring at the time of adoption, there were additional littermates present on the last occasion that we entered the nest. Females never adopted more than one orphan, and doing so would have made the costs of adoption outweigh the indirect benefits ( Table 1 ). 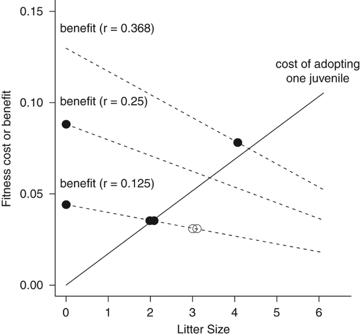Figure 2: Adoptions increase inclusive fitness, consistent with Hamilton's rule. Predicted fitness cost (solid line) of adoption to the surrogate dam increases, while fitness benefit (dash line) to the adopted juvenile decreases with litter size. Dashed lines represent three different degrees of relatedness calculated from a maternal pedigree or microsatellite allele frequencies and multiplied by the benefit to the juvenile (rb). Adoptions (closed circles) increased inclusive fitness, whereas unadopted litters (open circles) would have reduced inclusive fitness if adopted. Figure 2: Adoptions increase inclusive fitness, consistent with Hamilton's rule. Predicted fitness cost (solid line) of adoption to the surrogate dam increases, while fitness benefit (dash line) to the adopted juvenile decreases with litter size. Dashed lines represent three different degrees of relatedness calculated from a maternal pedigree or microsatellite allele frequencies and multiplied by the benefit to the juvenile ( rb ). Adoptions (closed circles) increased inclusive fitness, whereas unadopted litters (open circles) would have reduced inclusive fitness if adopted. Full size image Contrary to other documented cases of adoption by asocial species, adoptions by red squirrels in our study did not represent misdirected parental care, but rather a form of altruism that follows Hamilton's rule of kin selection. Studying an asocial species gave us a unique opportunity to calculate the fitness components of Hamilton's rule. We found that females did suffer fitness costs of adoption through reduced survival of their own juveniles, but this cost was offset by the inclusive fitness gained when the adopted juvenile was closely related. Further, although females had the opportunity to contravene Hamilton's rule by adopting unrelated juveniles or more than one related juvenile, they never did so. These results provide a particularly clear test of Hamilton's rule. Although the opportunity to increase inclusive fitness through adoption arises rarely (only 5 cases of adoption out of 2,230 litters), the clear bias towards adopting kin suggests that kin selection has been strong enough to favour the persistence of this unique behaviour. The mechanism by which female red squirrels assess their relatedness to juveniles or their dams is unknown and is a current focus of research at our study site. Although not specifically designed to study kin discrimination, previous cross-fostering experiments found that genetic and foster offspring grew at the same rate [9] , [19] , suggesting that female red squirrels do not differentially invest in genetic offspring and unrelated foster offspring present in their nest. This leads us to hypothesize that females assess relatedness of orphaned juveniles indirectly through recognition of their dam before her death, but this awaits experimental testing. Field methods Since 1989, we have studied red squirrels ( Tamiasciurus hudsonicus ) in Yukon, Canada, using complete enumeration to track the population size, survival and reproductive output of all females [12] , [20] . We repeatedly live trapped squirrels using Tomahawk traps and followed the pregnancy progression of all females through palpation and weight gain. Lactation or a sudden weight decrease indicated parturition, and we used behavioural observations and/or radio-telemetry to locate nests. We temporarily removed juveniles from their nests immediately after parturition to count, ear notch, weigh and determine the sex of each individual in the litter. We re-entered each nest at 25 days post-partum, when the juveniles were weighed again and given ear tags. Juveniles were then followed through observation and live trapping for as long as they were alive and remained in our study area [12] , [20] . Using these natal relationships, we constructed a complete maternal pedigree spanning multiple generations. Across 19 years (1989–2008), we monitored the survival and reproductive success of 6,793 juveniles in 2,230 litters produced by 1,101 free-ranging females. Cost/benefit analysis We constructed a general linear mixed-effects model for female ARS with litter size, litter size 2 , parturition date and juvenile growth rate as fixed effects. The quadratic term for litter size was added to investigate whether reproductive success was maximized at some intermediate litter size as a result of offspring size–number trade-offs (see below for results). ARS was measured as the number of juveniles born in the current year that survived up to the following spring (individuals are capable of breeding in the spring following their year of birth) using 753 observations by 502 females in 19 years. We only included control females that we knew had a single litter that year and for which we measured their date of parturition, litter size and offspring growth rate. Previous analyses found that these variables significantly influenced female ARS (for example, see McAdam and Boutin [19] and Réale et al . [21] ). Parturition date and juvenile growth rate were standardized within grid–year combinations, and the intercept of the model was forced through zero to correspond to the biologically relevant model in which females who did not produce any juveniles had zero ARS. Grid–year combinations were also fitted as a random effect to account for non-independence of ARS within grid–years. As our goal was to estimate parameters for the influence of litter size on ARS, and not to make inferences regarding their significance, we fit a general linear mixed-effects model (Gaussian error distribution) using the lmer function [22] in R [23] , rather than a generalized linear mixed-effects model (Poisson error distribution), because of the complications of back-transforming predicted values based on parameters estimated on a transformed (that is, link) scale. In this model, litter size had a positive effect on ARS (parameter±1 s.e.m. ; b =0.39±0.06), but the quadratic term indicated that the rate of increase in ARS with litter size declined as litter size increased ( b =−0.04±0.01). This relationship can also be visualized as a decline in the probability of each individual offspring surviving until spring as litter size increased ( Fig. 2 ). These analyses of long-term observational data are supported by previous experimental litter augmentations, which reduced juvenile survival, but did not decrease maternal survival or future reproductive success [9] . We calculated the predicted survival probability ( P x ) for individual offspring within a litter of size x as the predicted ARS for a litter of size x divided by litter size. We defined the fitness cost to the adopting female to be the difference between the probability of each juvenile surviving up to spring based on her natal litter size ( P x ) and the probability of survival based on her new litter size ( P x+1 ) multiplied by the number of juveniles in her natal litter ( x ) and her degree of relatedness to her offspring (0.5). The fitness benefit to the juvenile of being adopted was the probability that the adopted juvenile would survive to the following spring ( P x+1 ), where x represents the natal litter size of the surrogate female. We then calculated the minimum relatedness between the adopting female and the adopted juvenile that would be required for the benefits (discounted by r ) to exceed the costs of adopting according to Hamilton's rule ( Fig. 2 ) [2] . Here, we have calculated the costs and benefits of adoption based on ARS and have not considered costs of adoption reflected in the survival of the adopting female or her future reproductive success. Previous analyses have indicated that future breeding success is unaffected by previous breeding history, and that survival costs of reproducing compared with not-reproducing are restricted only to yearling females and females 6 years of age or older [24] . Furthermore, these survival costs of reproducing are independent of how many juveniles are reared at the time of weaning [24] . Surrogate females only adopted a single juvenile even though multiple juveniles were likely available to be adopted at the time they were orphaned (with the exception of case A4). The costs of adopting two juveniles were large enough to decrease inclusive fitness in five of the seven potential adoption cases ( Table 1 ). How to cite this article: Gorrell, J.C. et al . Adopting kin enhances inclusive fitness in asocial red squirrels. Nat. Commun. 1:22 doi: 10.1038/ncomms1022 (2010).